Visualizing specific protein glycoforms by transmembrane fluorescence resonance energy transfer Analyses of mice lacking glycosyltransferase have suggested that their pathological phenotypes are not attributable to the overall change of the sugar modification, but instead the result of changes of the glycan structures on a specific 'target' glycoprotein. Therefore, detecting or monitoring the glycosylation status of a specific protein in living cells is important, but no such methods are currently available. Here we demonstrate the detection of glycoforms of a specific glycoprotein using the fluorescence resonance energy transfer technique. Using model proteins, we detect characteristic fluorescence resonance energy transfer signals from the specific glycoform-bearing target glycoprotein. We also show that, upon insulin removal, sialylated glycoforms of green fluorescent protein-tagged GLUT4 seem to be internalized more slowly than non-sialylated GLUT4. This novel analytical imaging tool allows studying the roles of specific glycan modifications of a protein of interest. Glycosylation of proteins greatly influences physicochemical properties, such as solubility or thermal stability, as well as physiological properties, such as bioactivities or intracellular and intercellular trafficking. Metabolic sugar engineering, which inserts 'tags' into cellular glycoconjugates, has proven to be a powerful tool for the glycoproteomic analysis of a specific sugar modification [1] , [2] , [3] . This technique involves the incorporation of chemically modified sugars, such as azide- or alkyne-modified sugars, into cellular glycans via a normal biosynthetic pathway, and its subsequent detection with a probe, such as a FLAG-tag, biotin or fluorescent molecules [4] , [5] , [6] . Furthermore, application of this method for imaging of specific sugars in living cells and organisms has provided insights into the spatiotemporal expression and trafficking of glycans [7] , [8] , [9] , [10] . On the other hand, the currently available techniques face certain technical limitations, including the lack of selectivity, that is, there is no established method to detect a 'glycoform' (a protein with a specific glycan modification) of a given glycoprotein. However, in-depth analyses of the pathological phenotypes of several mice lacking glycosyltransferases have revealed that their phenotypes do not arise from the additive effects of the overall glycosylation change of many glycoproteins, but instead are caused by changes of the glycans on a specific 'target' glycoprotein [11] , [12] , [13] , [14] , [15] , [16] , [17] , [18] . Developing a method for the analysis of a specific glycoform of a target glycoprotein is therefore important, because one cannot currently carry out analyses until the glycoform has been biochemically isolated. To overcome this problem, we attempted to visualize the specific glycoforms of a protein of interest using an intramolecular fluorescence resonance energy transfer (FRET) technique. For this purpose, the target protein was tagged with green fluorescent protein (GFP) and a recently developed metabolic labelling method was used for sugar visualization. Although transmembrane FRET has not yet been rigorously exploited, to the best of our knowledge, the distance between the intracellular GFP of labelled proteins and the extracellular sialylated sites was estimated to be within the energy-transfer distance. Therefore, we examined whether specific FRET signals could be observed using model glycoproteins that monitor specific glycoforms. Intramolecular FRET signals were clearly detected, despite the fact that the two fluorophores on the protein (GFP) and sugar (tetramethylrhodamine (TMR) or Alexa Fluor 555) were segregated by a lipid bilayer. Using GLUT4-GFP (GFP-tagged GLUT4 glucose transporter) as a model substrate, we confirmed the observation of specific FRET signals that could be clearly distinguished from the background level (that is, intermolecular FRET with adjacent molecules or bleed-through of GFP signals). Analyses using total internal reflectron fluorescence (TIRF) microscopy demonstrated that sialylated GLUT4-GFP (FRET signals) appeared to be internalized at a slower rate than overall GLUT4 (GFP signals). This real-time imaging method will thus provide a novel powerful tool to analyse for a protein of interest the molecular details of glycan-based changes in various cellular events, such as intracellular/intercellular trafficking or cell surface stability. FRET-based imaging of sialylation of the target protein Although the recent technical development of a specific glycan-tagging system has proven to be a powerful tool, this method will label all glycoproteins bearing the modified sugars. Therefore, analysis of a specific glycoprotein with the labelled sugar is not possible, unless the protein of interest is isolated through laborious biochemical purification. In particular, the current technology does not allow monitoring a specific glycoform of a protein with an imaging technique. Trying to overcome these technical limitations, we combined the currently available sugar-labelling technique with GFP, a widely used fluorescent tag for proteins [19] , to establish a method for the detection of glycoforms of a specific glycoprotein. The rationale behind the idea is that if sugars can be labelled with a fluorescent probe that can be designed to be an acceptor for emission fluorescence released by GFP, we may be able to detect the glycoforms in a specific manner as intramolecular FRET signals ( Fig. 1 ). 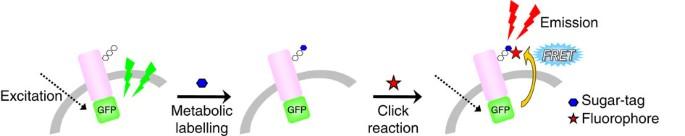Figure 1: FRET-based imaging of the glycosylation pattern of a specific glycoprotein. The strategy for visualization of a specific sugar on a target glycoprotein is shown. Glycans are metabolically labelled with azide sugars and click chemistry, and the target protein is conjugated with GFP. The specific glycoprotein can be visualized by FRET between GFP and the glycan-conjugated fluorophore. Figure 1: FRET-based imaging of the glycosylation pattern of a specific glycoprotein. The strategy for visualization of a specific sugar on a target glycoprotein is shown. Glycans are metabolically labelled with azide sugars and click chemistry, and the target protein is conjugated with GFP. The specific glycoprotein can be visualized by FRET between GFP and the glycan-conjugated fluorophore. Full size image We adopted an azide sugar (Ac 4 ManNAz) for fluorescence labelling of sialic acids in CHO-K1 or HeLa cells ( Supplementary Fig. S1 for the effect of Ac 4 ManNAz concentration on growth and toxicity to HeLa cells). Ac 4 ManNAz was found to be incorporated into cells as sialic acids, because the fluorescent signals were completely abolished by prior treatment of cells with sialidase ( Supplementary Fig. S2 ). SiaNAz, an azide-tagged sialic acid, was labelled with a fluorescent tag using TMR alkyne. The labelling reaction was carried out in fixed non-permeabilized cells, such that only the cell surface sialic acids could be labelled. To confirm the cell fixation, GLUT4-GFP was used. All the GFP tags on GLUT4 were found to reside in the cytosol, based on flow cytometric analysis ( Supplementary Fig. S3a ), suggesting the uniform orientation (topology) of this protein. We confirmed that the cells were not permeabilized under our fixation conditions, because an anti-GFP antibody was unable to access the GFP tags unless a detergent such as Triton X-100 was used for permeabilization ( Supplementary Fig. S3b ). Sialylation and FRET imaging of EGFR Having confirmed the glycan labelling, we expressed epidermal growth factor receptor (EGFR)–GFP as a model glycoprotein to examine whether we could detect FRET signals between the GFP-tagged and TMR-labelled sialic acids. EGFR is a single transmembrane protein bearing 12 N -glycosylation sites with various glycan structures [20] , and therefore, labelling of glycans with multiple TMR sialic acids was expected. EGFR–GFP was expressed in CHO-K1 cells, as well as in control Lec2 cells that lack sialylation owing to a defect in CMP-Sia transporter activity [21] . As shown in Fig. 2a–d , EGFR–GFP was expressed efficiently in both CHO-K1 and Lec2 cells. Without EGFR–GFP, no FRET signals were observed ( Fig. 2a ). After the sialic acids were labelled with TMR, FRET was only detected in CHO-K1 cells ( Fig. 2c ) and not without Ac 4 ManNAz treatment ( Fig. 2b ), or in Lec2 cells ( Fig. 2d ). These results collectively indicated that the FRET signals did not arise from bleed-through of GFP fluorescence, but from TMR-labelled SiaNAz. Moreover, the emission spectrum of the cells shown in Fig. 2c (CHO-K1, EGFR–GFP plus SiaNAz–TMR) at 488-nm excitation clearly showed a second peak at around 580 nm, together with the major peak at around 510 nm ( Fig. 2e , spectrum c). The second peak was significantly higher than that observed without the EGFR–GFP expression ( Fig. 2e , spectrum a), even when the spectra were normalized by the degree of TMR labelling ( Supplementary Fig. S4 ), further suggesting that the observed signals did indeed come from FRET. Taking all these results together, we demonstrated successful energy transfer from GFP to TMR using EGFR–GFP as a model protein. 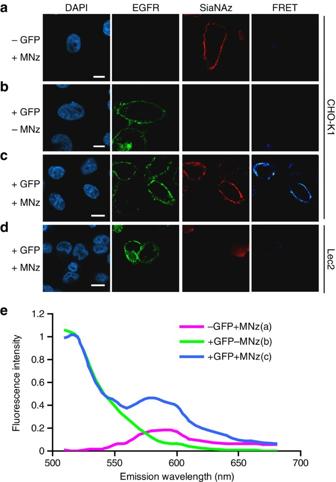Figure 2: FRET imaging of sialylated EGFR. (a–d) Fluorescence images of the sialylated glycoform of EGFR. Control CHO-K1 cells (a), EGFR–GFP-transfected CHO-K1 cells (b,c) and Lec2 mutant cells (d) were incubated with (a,c,d) or without (b) 50 μM Ac4ManNAz (MNz) and labelled with TMR alkyne. Nuclei: DAPI (4′,6-diamidino-2-phenylindole; blue), EGFR: GFP (green), SiaNAz: TMR (red), SiaNAz-bearing EGFR: FRET (pseudo). Scale bar equals 10 μm. (e) Emission spectra obtained from panelsa–cwhen excited at 488 nm. The second peak around 580 nm in panelcrepresents the FRET signal, which is well above the background level (observed in the absence of GFP, panela). Figure 2: FRET imaging of sialylated EGFR. ( a – d ) Fluorescence images of the sialylated glycoform of EGFR. Control CHO-K1 cells ( a ), EGFR–GFP-transfected CHO-K1 cells ( b , c ) and Lec2 mutant cells ( d ) were incubated with ( a , c , d ) or without ( b ) 50 μM Ac 4 ManNAz (MNz) and labelled with TMR alkyne. Nuclei: DAPI (4′,6-diamidino-2-phenylindole; blue), EGFR: GFP (green), SiaNAz: TMR (red), SiaNAz-bearing EGFR: FRET (pseudo). Scale bar equals 10 μm. ( e ) Emission spectra obtained from panels a – c when excited at 488 nm. The second peak around 580 nm in panel c represents the FRET signal, which is well above the background level (observed in the absence of GFP, panel a ). Full size image Intramolecular FRET is observed between GLUT4 and SiaNAz Although FRET signals were detected using EGFR, the issue of whether the signals came from intramolecular FRET on the same protein remained to be clarified, because the signals may have been derived from the TMR-labelled sugars on adjacent molecules. To clarify this issue, we used another model substrate, GLUT4, because it only contains a single N -glycosylation site at Asn 57 and the specificity of FRET can be evaluated using a mutant lacking this sole glycosylation site (N57Q) [22] ( Fig. 3a ). We expressed wild-type GLUT4-GFP (WT) and its glycosylation mutant GLUT4 (N57Q)-GFP (N57Q) in HeLa cells. It was previously demonstrated that WT is capable of responding to insulin treatment, whereas N57Q loses this insulin responsiveness, when expressed in HeLa cells, thereby underscoring the importance of the sole N -glycan on this protein [22] . We found that the structure of the N -glycan on GLUT4 was not uniform, being a mixture of both non-sialylated and sialylated glycans ( Supplementary Fig. S5 ). As shown in Fig. 3b , FRET signals were observed for GLUT4 when WT was expressed in the presence of Ac 4 ManNAz (upper panel). In sharp contrast, FRET signals were not observed when N57Q was expressed (lower panel), despite the fact that the mutant is expressed well in HeLa cells [22] . These results clearly suggested that the FRET signals between GLUT4-GFP and SiaNAz–TMR observed in WT came from the same molecule (that is, intramolecular FRET on GLUT4 or FRET between two GLUT4 molecules), and not from the sugars on adjacent proteins, because such signals would also be observed using N57Q. Specific FRET signals were also obtained when WT or N57Q was expressed in CHO-K1 cells ( Supplementary Figs S6 and S7 ). 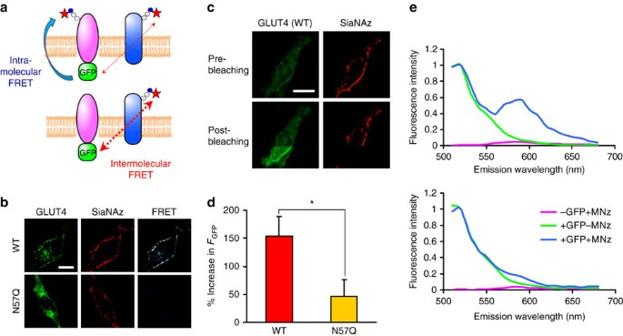Figure 3: FRET imaging of sialylated GLUT4-GFP. (a) Schematic model of intramolecular and intermolecular FRET in cells expressing GLUT4 (WT)-GFP (upper) or GLUT4 (N57Q)-GFP (lower). (b) Fluorescence images of HeLa cells transfected with WT or N57Q, treated with 50 μM Ac4ManNAz, and labelled with TMR alkyne to visualize SiaNAz. GLUT4: GFP (green), SiaNAz: TMR (red), SiaNAz-bearing GLUT4: FRET (pseudo). Scale bar equals 20 μm. (c) Acceptor photobleaching. Scale bar equals 20 μm. (d) Average increases in the donor (GFP) fluorescence at the cell surface after TMR photobleaching using WT and the glycosylation mutant N57Q. Data are mean±s.d. (n=5). Data were statistically analysed by Student'st-test (*P<0.001). (e) Emission spectra of WT (upper) and N57Q (lower) with 488-nm excitation. Figure 3: FRET imaging of sialylated GLUT4-GFP. ( a ) Schematic model of intramolecular and intermolecular FRET in cells expressing GLUT4 (WT)-GFP (upper) or GLUT4 (N57Q)-GFP (lower). ( b ) Fluorescence images of HeLa cells transfected with WT or N57Q, treated with 50 μM Ac 4 ManNAz, and labelled with TMR alkyne to visualize SiaNAz. GLUT4: GFP (green), SiaNAz: TMR (red), SiaNAz-bearing GLUT4: FRET (pseudo). Scale bar equals 20 μm. ( c ) Acceptor photobleaching. Scale bar equals 20 μm. ( d ) Average increases in the donor (GFP) fluorescence at the cell surface after TMR photobleaching using WT and the glycosylation mutant N57Q. Data are mean±s.d. ( n =5). Data were statistically analysed by Student's t -test (* P <0.001). ( e ) Emission spectra of WT (upper) and N57Q (lower) with 488-nm excitation. Full size image To further address the intramolecular FRET signals observed in Fig. 3b in a more convincing manner, we carried out acceptor photobleaching experiments to confirm the enhanced emission fluorescence of GFP after bleaching of the acceptor (TMR) fluorescence. As shown in Fig. 3c , a portion of the cells was exposed to a maximal laser light at 559 nm to bleach the fluorescence of TMR. Subsequently, direct emission from the donor (GFP) was found to be increased as a consequence of preventing FRET through the acceptor photobleaching. The mean value of the increased GFP fluorescence for WT was significantly higher than that for N57Q ( Fig. 3d ), further indicating that the detected FRET signals were mostly derived from intramolecular FRET. On the basis of the data in Fig. 3d , the overall FRET efficiencies of WT and N57Q estimated from the acceptor photobleaching results were 0.60 and 0.28, respectively; and based on these values, and considering the fact that N57Q does not have intramolecular FRET, the intramolecular FRET efficiency between WT and SiaNAz–TMR on GLUT4 was estimated to be 0.52. Moreover, when the fluorescence emission spectrum of WT labelled with SiaNAz–TMR under excitation at 488 nm was compared with that of N57Q, WT showed a clear FRET peak at around 580 nm, whereas the spectrum for N57Q was much more depressed around the emission wavelength of TMR ( Fig. 3e ). Taking all these findings together, it was clearly demonstrated that intramolecular FRET could be detected in a specific manner between GLUT4-GFP and SiaNAz–TMR on GLUT4. FRET signals were also observed for GLUT4-GFP when alkynylated fucose, an analogue of fucose, was used for labelling of sugars ( Supplementary Fig. S8 ). Consistent with a previous report [6] , however, it required a much higher concentration of the analogue. Time-lapse imaging of sialylated GLUT4 using FRET GLUT4 is known to change its subcellular localization from intracellular vesicles to the cell surface in response to insulin treatment [23] , [24] , [25] . Therefore, we wanted to be able to monitor the movement of the sialylated forms of GLUT4, that is, the FRET signals from GLUT4-GFP. Again, labelling was carried out under non-permeabilized conditions using fixed HeLa cells, so that only the cell surface sialic acids, and not the intracellular ones, could be labelled with TMR. Upon insulin treatment, the cell surface expression of GLUT4 was enhanced in HeLa cells ( Supplementary Fig. S9a , compare upper and middle GLUT4 panels), as reported previously [22] . Clear FRET signals were observed for WT treated with Ac 4 ManNAz ( Supplementary Fig. S9a , middle panel), whereas little signalling was detected for N57Q ( Supplementary Fig. S9a , lower panel). Along with the increased cell surface expression of WT, the FRET signals on the cell surface were also greatly enhanced, whereas no such enhancement was observed for N57Q ( Supplementary Fig. S9b ). These results support the previous finding that the N -glycan of GLUT4 is important for its responsiveness to insulin treatment [22] . Next, we examined whether the FRET signals could be utilized for time-lapse experiments to track the movement of glycoforms of GLUT4 (sialylated GLUT4). To this end, a reagent developed by Boons and colleagues [26] , [27] was used, because it can react with azide groups under copper-free conditions and is therefore compatible with live-cell imaging. We conjugated Alexa Fluor 555 with this azide-reactive compound for the labelling of SiaNAz (DIBO-555). We monitored the movement of GLUT4 and the FRET signals by time-lapse experiments ( Fig. 4 ). We chose 37 °C for 5 min to label the cells to minimize the labelling of SiaNAz inside the cells. Although cell-surface-specific labelling was also observed by labelling at 4 °C for 60 min ( Supplementary Fig. S10 ), we decided not to use these conditions to avoid the problem of defocusing upon raising the temperature to 37 °C. Under this condition, the endocytosed fluorescence (SiaNAz) was found to be comparable with the condition at 4 °C for 60 min ( Supplementary Fig. S11 ). GLUT4-GFP was first accumulated at the cell surface by insulin treatment, and then cell surface SiaNAz was labelled in living cells. Under these conditions, FRET signals were hardly detected inside the cells ( Fig. 4 , lower left panel). Internalization was initiated by removal of the insulin, and the movement of the FRET signals (sialylated GLUT4) was monitored by time-lapse analysis. Significant incorporation of the FRET signals into intracellular dots was observed. These findings support our idea that, as long as proper controls are included, the movement of intramolecular FRET signals derived from sialylated GLUT4 can be monitored by time-lapse imaging. 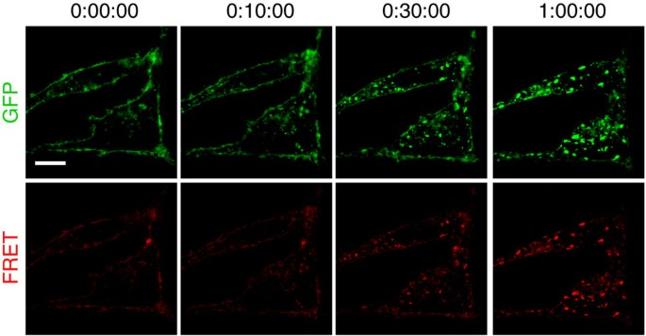Figure 4: Time-lapse imaging of sialylated GLUT4-GFP. HeLa cells transfected with GLUT4-GFP were treated with 100 μM Ac4ManNAz, serum-starved, stimulated with insulin, and then labelled with DIBO-555 at 37 °C for 5 min. The cells were monitored by confocal microscopy. The time (h:min:s) is indicated at the top of each image. Images are representative of 10 different visual fields. Scale bar equals 10 μm. Figure 4: Time-lapse imaging of sialylated GLUT4-GFP. HeLa cells transfected with GLUT4-GFP were treated with 100 μM Ac 4 ManNAz, serum-starved, stimulated with insulin, and then labelled with DIBO-555 at 37 °C for 5 min. The cells were monitored by confocal microscopy. The time (h:min:s) is indicated at the top of each image. Images are representative of 10 different visual fields. Scale bar equals 10 μm. Full size image GLUT4 internalization may be distinct between glycoforms To evaluate the internalization kinetics of sialylated GLUT4 with this FRET technique, we used TIRF microscopy. In TIRF, only fluorophores very close (for example, within ~100 nm) to the coverslip–sample interface are excited, thereby allowing the detection of events adjacent to the plasma membrane [28] . This method has been used for analyses of intracellular trafficking of GLUT4 proteins [23] , [29] , [30] . However, when we attempted live-cell imaging by TIRF, we were unable to chase the GLUT4 movement because TIRF can only monitor a single cell in a single analysis, and it was not possible to choose cells responding properly to insulin in advance. Therefore, we used fixed cells for the TIRF analysis. Again, cells expressing GLUT4-GFP were treated with insulin to allow GLUT4 to become localized at the cell surface at the maximal level. The cell surface SiaNAz was then labelled in living cells, and internalization was initiated by removal of the insulin. Therefore, most, if not all, of the vesicles observed by TIRF in this experiment should represent those just internalized from the cell surface. Cells fixed at the indicated time points were subjected to the TIRF analysis. Consistent with previous reports, dotted signals from GFP (GLUT4) and its FRET signals (Sia-GLUT4) were detected by TIRF imaging ( Fig. 5a , left and middle panels). It should be noted that the FRET signal intensities were not proportional to those of GFP (right panel), suggesting that the signals were specific and not merely bleed-through of the GFP fluorescence. 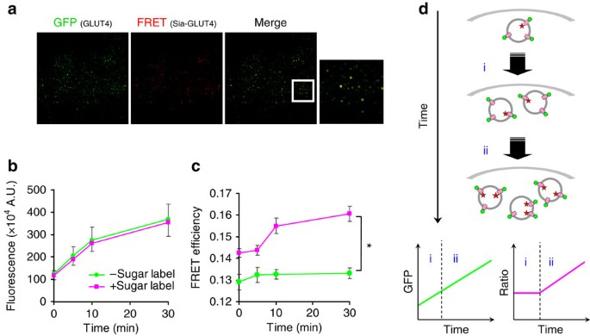Figure 5: Internalization analysis of sialylated GLUT4 using TIRF microscopy. (a) TIRF images showing the distributions of GLUT4 (WT)-GFP and SiaNAz-bearing GLUT4-GFP. The right image is a magnification of the marked region in the merged image. (b,c) GLUT4 (WT)-GFP-transfected HeLa cells were treated with 100 μM Ac4ManNAz, serum-starved, stimulated with insulin, and then incubated with or without DIBO-555 at 37 °C for 5 min. The cells were incubated in KRB for 5, 10 or 30 min, and then fixed. –Sugar label: samples without DIBO-555 labelling, +sugar label: samples with DIBO-555 labelling. The dot intensities in the GFP channels (b) and the FRET efficiencies (c) were analysed in 10 different cells, and the data represent mean±s.e.m. Data were statistically analysed by Student'st-test (*P<0.001). (d) Schematic models of GLUT4 internalization kinetics. When the internalization rate does not change between sialylated GLUT4 and overall GLUT4, the FRET efficiency (ratio of FRET/GFP signals) will remain constant at each time point (stage i). On the other hand, increased FRET signals were observed after 5 min, suggesting that more sialylated GLUT4 species were internalized at later time points (stage ii). Figure 5: Internalization analysis of sialylated GLUT4 using TIRF microscopy. ( a ) TIRF images showing the distributions of GLUT4 (WT)-GFP and SiaNAz-bearing GLUT4-GFP. The right image is a magnification of the marked region in the merged image. ( b , c ) GLUT4 (WT)-GFP-transfected HeLa cells were treated with 100 μM Ac 4 ManNAz, serum-starved, stimulated with insulin, and then incubated with or without DIBO-555 at 37 °C for 5 min. The cells were incubated in KRB for 5, 10 or 30 min, and then fixed. –Sugar label: samples without DIBO-555 labelling, +sugar label: samples with DIBO-555 labelling. The dot intensities in the GFP channels ( b ) and the FRET efficiencies ( c ) were analysed in 10 different cells, and the data represent mean±s.e.m. Data were statistically analysed by Student's t -test (* P <0.001). ( d ) Schematic models of GLUT4 internalization kinetics. When the internalization rate does not change between sialylated GLUT4 and overall GLUT4, the FRET efficiency (ratio of FRET/GFP signals) will remain constant at each time point (stage i). On the other hand, increased FRET signals were observed after 5 min, suggesting that more sialylated GLUT4 species were internalized at later time points (stage ii). Full size image To determine whether sugar labelling affects the efficiency of GLUT4 internalization, we first detected the total intensities of dots from the GFP channel in both sugar-labelled (+sugar label) and sugar-unlabelled (−sugar label) cells. The kinetics of GFP internalization was found to be quite similar with or without DIBO-555 labelling, clearly indicating that the internalization of GLUT4-GFP was not affected by the sugar labelling with the Alexa 555-conjugated reagent ( Fig. 5b ). As the TIRF analysis only captured vesicles just inside the cell surface, we observed 'snapshots' of GLUT4-containing vesicles, mostly internalized from the cell surface under our experimental conditions, at each time point. If the internalization rate did not alter between sialylated GLUT4 and overall GLUT4, the FRET efficiency (ratio of FRET/GFP signals) would remain constant at each time point. On the other hand, our results indicated that increased FRET signals were observed after 5 min ( Fig. 5c ). These results suggested that more sialylated glycoforms were observed by TIRF at later time points, indicating slower internalization kinetics of the sialylated GLUT4 species ( Fig. 5d ). These observations may suggest that the sialylated form of GLUT4 shows relatively slow internalization compared with non-sialylated GLUT4. In this study, we successfully developed a novel method to detect the glycoforms of a protein of interest using a FRET technique. This simple idea may have been underappreciated on the basis of the assumption that the tags are often segregated by the lipid bilayer ( Fig. 1 ) and therefore, too far away from one another to observe the FRET signals. However, the thickness of the lipid bilayer is around 30 Å [31] , and the thickness of GLUT4, one of our model proteins, appears to be around 40 Å [32] . FRET has been observed when the donor and acceptor molecules are as far apart as 100 Å [33] , [34] . Moreover, the distance at which energy transfer from enhanced GFP to Alexa Fluor 555 shows 50% efficiency ( R 0 ) is estimated to be 63 Å ( http://www.invitrogen.com/site/us/en/home/References/Molecular-Probes-The-Handbook/Technical-Notes-and-Product-Highlights/Fluorescent-Probes-for-Use-with-GFP.html ). These facts led us to believe that FRET segregated by a lipid bilayer is indeed an achievable goal. In this study, we used two model proteins (EGFR and GLUT4) and showed that the FRET signals were strong enough for detection. In particular, for GLUT4 bearing only a single N -glycan, the sialylated forms were detected in a highly specific manner, and a non-glycosylated mutant did not give detectable FRET signals even in the presence of labelled sugars. These results collectively indicate that most, if not all, of the FRET signals should be derived from intramolecular FRET. However, to utilize this technique for proteins that form complexes, precautions need to be taken to evaluate whether the detected signals are coming from intramolecular FRET or from FRET between adjacent molecules, such as other components in the complex. Therefore, appropriate controls are imperative. It also remains to be determined whether the positions of N -glycans can affect the efficiency of FRET. It should be noted here that our technique only allows the detection of several different glycoforms containing a specific sugar, and that imaging a specific glycoform, that is, a protein with a specific glycan structure, is not currently possible. In the future, however, the development of sugar analogues that can act as a substrate for a specific glycosyltransferase will allow us to achieve the detection of more specific glycoforms. Recent progress in protein tagging has allowed us to use different techniques to label proteins in vivo [35] , [36] . Such techniques will enable us to minimize the sizes of the tags and also potentially overcome the distance problem, because a tag can potentially be placed in proximity to the glycosylation site. We showed that not only sialic acids, but also fucose, could be successfully used for FRET detection. These findings open up the possibility of further applications of this FRET technique, such as simultaneous detection of different glycoforms on the same protein using, for example, a double FRET technique to detect two FRET pairs sharing one fluorophore [37] , [38] , [39] . Our analysis of the sialylated glycoform of GLUT4 indicated that different kinetics might be involved in its internalization depending on the glycan structure. Although such glycan-dependent changes in the turnover of cell surface proteins have been demonstrated in a number of studies [15] , [16] , [17] , [18] , they all relied on knock-out mice or cell lines for glycosyltransferases, making it impossible to completely exclude the indirect effects of other proteins that also receive altered glycosylation. In our imaging analysis, on the other hand, a clear difference in the internalization kinetics between the sialylated form (FRET) and the overall protein (GFP) was observed without any specific defects in the glycosylation pathway. These phenomena could be explained by the existence of a mechanism for retaining sialylated glycoproteins by a lectin-based lattice [18] or equivalent, although the molecular details remain to be determined. Regardless of the mechanism, our study opens up a way to analyse the different kinetics of the movements of distinct glycoforms using an imaging technique. The use of real-time imaging analysis will be particularly attractive, because biochemical techniques can only show the steady-state conditions of the glycoforms. The importance of glycans in various cellular events, especially intracellular and intercellular trafficking of proteins, has been shown by numerous studies, and FRET analysis of glycoforms of a target protein should provide another valuable tool for in-depth analyses of the roles of glycans. Microscopic analysis and FRET measurement Cells were grown on cover glasses (12-mm diameter) placed in 24-well plates in appropriate medium with or without 50 μM Ac 4 ManNAz or 500 μM fucose alkyne for 2 days. The cells were washed with PBS, fixed with 3% paraformaldehyde in PBS for 20 min, washed twice with PBS and blocked with 3% bovine serum albumin in PBS for 30 min. Subsequently, the cells were subjected to the probe-labelling reaction using Click-iT Protein Analysis Detection Kits (Molecular Probes), essentially according to the manufacturer's protocol. Briefly, 1 μM TMR alkyne (for SiaNAz detection) or 5 μM TMR azide (for fucose-alkyne detection) in 250 μl of click reaction solution (10 μl of Click-iT reaction buffer (component A), 2 μl of CuSO 4 solution (component B), 4 μl of component C, 4 μl of component D and 230 μl of PBS) was prepared, and fixed cells were subjected to the click reaction for 30 min at room temperature. The cells were then washed, mounted with a drop of Vectashield (Vector Laboratories) and observed by laser scanning confocal microscopy (Olympus FV500). Lambda scanning was performed using a Leica TCS SP2. To measure FRET, the samples were excited at 488 nm, and the fluorescence intensities of the donor (GFP) and acceptor (TMR) were measured using an appropriate filter set. Image processing was performed with MetaMorph software (Molecular Devices). Acceptor photobleaching was carried out using an FV1000 laser scanning confocal microscope (Olympus). Basal images of GLUT4-GFP and SiaNAz–TMR were acquired first. A portion of the cells was then exposed to maximal-intensity laser light at 559 nm to bleach the TMR. The average increases in the donor (GFP) fluorescence at the cell surface after TMR photobleaching were measured using the MetaMorph software. The efficiency of energy transfer ( E ) was given by the following equation: [40] E =1− F DA / F D = k T /( k D + k T ), where F D and F DA are the relative fluorescence intensities of the donor in the absence ( F D ) or presence ( F DA ) of the acceptor, k D is the decay rate of the donor in the absence of the acceptor, and k T is the energy-transfer rate. As the FRET signals observed in WT may contain both intermolecular and intramolecular FRET, the FRET efficiency for WT can be described as E wt =( k intra +k inter )/( k D +k inter +k intra )=1− k D /( k D +k inter +k intra ). On the other hand, the FRET signals in N57Q are only derived from intermolecular FRET between GFP and SiaNAz on the adjacent molecules, and therefore, the efficiency is given by E N57Q = k inter /( k D +k inter )=1− k D /( k D +k inter ). On the basis of the data shown in Fig. 3d , E WT was 0.60 and E N57Q was 0.28. Accordingly, the intramolecular FRET efficiency was calculated as E WT(intra) = k intra /( k D + k intra )=0.52. Time-lapse imaging of living cells Experiments were carried out using an FV1000-D (Olympus) equipped with an incubator to keep the cells at 37 °C throughout the experiments. HeLa cells expressing GLUT4-GFP were seeded onto a glass-bottom dish (35-mm diameter) in appropriate medium with or without 100 μM Ac 4 ManNAz for 2 days. Before the imaging experiments, the cells were serum-starved in Krebs–Ringer bicarbonate (KRB) buffer (129 mM NaCl, 4.7 mM KCl, 1.2 mM KH 2 PO 4 , 5 mM NaHCO 3 , 10 mM HEPES, 3 mM D -glucose, 2.5 mM CaCl 2 , 1.2 mM MgCl 2 and 0.2% bovine serum albumin; pH adjusted to 7.4 with NaOH) with or without 100 μM Ac 4 ManNAz for 3 h. GLUT4-GFP-expressing cells were then stimulated with insulin (100 nM) for 30 min, and SiaNAz was subsequently labelled with 50 μM DIBO-555 for 5 min at 37 °C. After washing, images of the cells in KRB buffer were acquired at 5-min intervals at 37 °C under 5% CO 2 . TIRF-imaging collection and analysis TIRF images were acquired using an EM-CCD camera (ImagEM; Hamamatsu) attached to a TIRF microscope, based on an IX-81 inverted microscope (Olympus) equipped with a ×60 NA 1.45 oil-immersion objective (PlanApo; Olympus). Dual-colour TIRF images were acquired with excitation at 488 nm, and emissions at 500–550 nm for GFP and 568–613 nm for FRET. The experiments were performed at 37 °C. HeLa cells expressing GLUT4-GFP were cultured with 100 μM Ac 4 ManNAz on a glass-bottom dish, and serum-starved as described above. The cells were then stimulated with insulin (100 nM) for 30 min. Subsequently, SiaNAz was labelled with 50 μM DIBO-555 for 5 min at 37 °C. After washing, the cells in KRB buffer were incubated and fixed with methanol at various time points. Images were collected for both the GFP and FRET channels. The background was subtracted from the fluorescence images in the GFP channel using the median filter of the MetaMorph software. Dot positions were determined by setting the threshold for each image. The positions were then transferred to the corresponding image in the FRET channel, and the green and red pixel intensities were logged. The FRET efficiency was calculated as red pixel intensities/green pixel intensities. How to cite this article: Haga, Y. et al . Visualizing specific protein glycoforms by transmembrane fluorescence resonance energy transfer. Nat. Commun. 3:907 doi: 10.1038/ncomms1906 (2012).